Orbital reconstruction in nonpolar tetravalent transition-metal oxide layers A promising route to tailoring the electronic properties of quantum materials and devices rests on the idea of orbital engineering in multilayered oxide heterostructures. Here we show that the interplay of interlayer charge imbalance and ligand distortions provides a knob for tuning the sequence of electronic levels even in intrinsically stacked oxides. We resolve in this regard the d -level structure of layered Sr 2 IrO 4 by electron spin resonance. While canonical ligand-field theory predicts g || -factors less than 2 for positive tetragonal distortions as present in Sr 2 IrO 4 , the experiment indicates g || is greater than 2. This implies that the iridium d levels are inverted with respect to their normal ordering. State-of-the-art electronic-structure calculations confirm the level switching in Sr 2 IrO 4 , whereas we find them in Ba 2 IrO 4 to be instead normally ordered. Given the nonpolar character of the metal-oxygen layers, our findings highlight the tetravalent transition-metal 214 oxides as ideal platforms to explore d -orbital reconstruction in the context of oxide electronics. Their unique diversity of transport and magnetic properties endows transition-metal (TM) oxides with a long-term potential for applications in microelectronics and electrical engineering. Nowadays the search for new or superior properties goes beyond known bulk phases and includes oxide interfaces and stacked superlattices [1] , [2] . As compared with the bulk material, at interfaces the modification of the nearby surroundings can significantly affect the valence electronic structure, in particular, the occupation of the d -shell levels [1] , [2] , [3] , [4] , [5] . This is often referred to as orbital reconstruction [3] , [4] , [5] and brings to the fore the most basic aspect in electronic-structure theory: how energy levels in quantum matter are formed and populated. A variety of intrinsically stacked crystalline oxides is presently known. The high-temperature cuprate superconductors [6] , for example, fall in this category but also iridates of the type A 2 IrO 4 (A=Sr 2+ , Ba 2+ ) that closely resemble undoped cuprates, both structurally and magnetically [7] , [8] , [9] , [10] , [11] . Sr 2 IrO 4 has a rather simple crystalline structure displaying stacked, quasi two-dimensional (2D) IrO 2 and double SrO layers. We shall demonstrate that in this system the occupation of the valence d electronic levels differs from what is expected in textbook ligand-field theory due to electrostatics that involves both types of metal-oxygen sheets. In particular, we show that, as compared with the isostructural cuprate La 2 CuO 4 , a different distribution of ionic charges between the TM-O 2 and A-O layers modifies the sequence of energy levels within the t 2g and e g manifolds and consequently very fundamental physical properties such as the magnetic g factors, which determine the relation between the magnetic moment and quantum number of a magnetic particle. Our findings are of direct relevance to the field of stacked oxide heterostructures and provide a guideline on how low-symmetry crystal fields at d -metal sites can be altered and potentially engineered through the appropriate design of successive ionic layers. To show this we first use electron spin resonance (ESR) measurements to untangle the 5 d -shell electronic structure of crystalline Sr 2 IrO 4 , in particular, the exact order of the Ir t 2g levels. The single s =1/2 hole present in these t 2g orbitals carries an angular moment l eff =1 and is subject to a large spin-orbit coupling (SOC), which in first approximation results in an effective Ir 4+ moment, or pseudospin, j eff = l eff − s ≈1/2 (refs 7 , 12 , 13 ). We compare the experimental properties of these pseudospins with the ones we have calculated by ab initio quantum chemistry methods. This combined approach, explored here on a strongly spin-orbit coupled material for the first time, provides direct access to the spatial anisotropies of the g factors and further to the detailed microscopic superexchange interactions. The ESR measurements and theory are found to agree on a quantitative level and moreover undoubtedly show that the d -level ordering in Sr 2 IrO 4 is inverted with respect to the normal ordering in the sister iridate Ba 2 IrO 4 or the isostructural 214 cuprate superconductors. The good agreement between the ESR data and the outcome of the computational methodology we describe and employ here establishes the latter as a reliable tool for the investigation of nontrivial electronic structures and magnetic couplings. Pseudospins and effective Hamiltonian Mott-Hubbard physics in d -metal compounds has been traditionally associated with first-series (3 d ) TM oxides. However, recently, one more ingredient entered the TM-oxide ‘Mottness’ paradigm—large SOC’s in 5 d systems. SOC in 5 d and to some extent 4 d anisotropic oxides modifies the very nature of the correlation hole of an electron, by admixing the different t 2g components [12] , [13] , changes the conditions for localization [7] , the criteria of Mottness and further gives rise to new types of magnetic ground states and excitations [9] , [11] . While various measurements indicate that indeed spin-orbit-coupled j eff ≈1/2 states form in A 2 IrO 4 (refs 7 , 9 , 14 ), it has been also pointed out that off-diagonal SOC’s may mix into the ground state (GS) wavefunction substantial amounts of character [15] , [16] , [17] , [18] . Such many-body interactions were shown to produce remarkable effects in X-ray absorption and X-ray magnetic circular dichroism (XMCD): the branching ratio between the L 3 and L 2 Ir 2 p absorption edges reaches values as large as 4, nearly 50% higher than the 2.75 value for a ‘pure’ j eff =1/2 system [19] . In addition, low-symmetry noncubic fields produce sizeable splittings of the 5 d t 2g levels, in some cases close to or even larger than ∼ 1/2 eV (refs 20 , 21 , 22 ), and therefore admix the j eff =1/2 and components [13] , [15] . The structure of the spin-orbit GS depends on both the strength and sign of these splittings. Interestingly, the best fits of the X-ray absorption and XMCD data are achieved in Sr 2 IrO 4 with a negative t 2g tetragonal splitting [19] , although the oxygen octahedra in this material display a distinct positive tetragonal distortion—the IrO 6 octahedra are substantially elongated [23] (a negative tetragonal splitting should occur when the IrO 6 octahedra are compressed [13] , [24] , see Fig. 1 ). This is already a first indication of the level inversion that our ESR measurements and quantum chemistry calculations show to take place in Sr 2 IrO 4 . 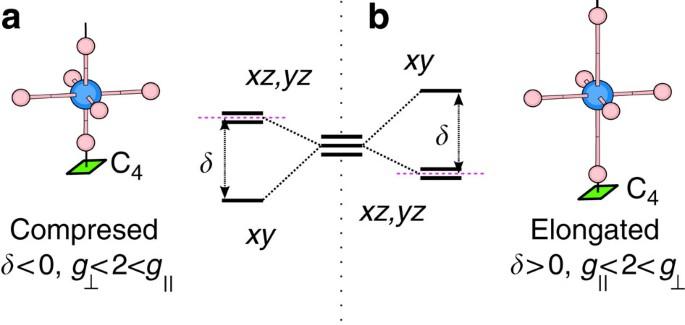Figure 1: TMt2gsplittings for tetragonal distortions of the oxygen octahedron sans SOC. (a)zaxis compression of the octahedron corresponds to a tetragonal splittingδ<0, causes an orbital dublet to be lowest in energy and thegfactors to be ordered as. (b) Elongation of the octahedron (δ>0) causes an orbital singlet to be lowest in energy and thegfactors to be ordered as. Purple dashed lines indicate the conventional zero level used to define the sign ofδ. Figure 1: TM t 2g splittings for tetragonal distortions of the oxygen octahedron sans SOC. ( a ) z axis compression of the octahedron corresponds to a tetragonal splitting δ <0, causes an orbital dublet to be lowest in energy and the g factors to be ordered as . ( b ) Elongation of the octahedron ( δ >0) causes an orbital singlet to be lowest in energy and the g factors to be ordered as . Purple dashed lines indicate the conventional zero level used to define the sign of δ . Full size image The interactions between a pair 〈 ij 〉 of nearest-neighbour (NN) 1/2 pseudospins in the presence of an external magnetic field h is given by the effective Hamiltonian where , are pseudospin ( j eff ≈1/2) operators, J is the isotropic Heisenberg exchange, D =(0,0, D ) defines the antisymmetric Dzyaloshinskii-Moriya (DM) coupling, is a symmetric traceless second-rank tensor describing the symmetric anisotropy and due to the staggered rotation of the IrO 6 octahedra the tensor splits for each of the two sites into uniform and staggered components (see for example, refs 16 , 25 ). This effective spin Hamiltonian is of direct relevance to the interpretation of the ESR data. ESR measurements For a single crystal of Sr 2 IrO 4 we observe antiferromagnetic resonance (AFR) modes in the sub-THz frequency domain [26] as displayed in Fig. 2 . 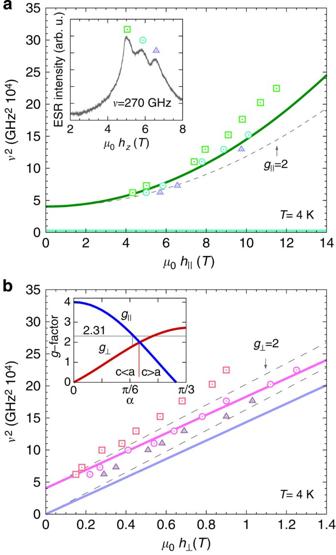Figure 2: ESR data for Sr2IrO4. (a) Out-of-plane magnetic-field geometries; the inset shows a representative AFR spectrum. (b) In-plane magnetic fields; the inset demonstrates theg-factor anisotropy as function of the tetragonal distortion parameterα(see text). Symbols denote experimental data points—solid lines are theoretical curves using equations (2, 3, 4) and the quantum chemically computedgfactorsg||=2.31,g⊥=1.76 (seeTable 1); dashed lines are calculated assuming isotropicgfactors. There are two modes if h || z : a gapless Goldstone mode v ||1 =0 and a gapped excitation Figure 2: ESR data for Sr 2 IrO 4 . ( a ) Out-of-plane magnetic-field geometries; the inset shows a representative AFR spectrum. ( b ) In-plane magnetic fields; the inset demonstrates the g -factor anisotropy as function of the tetragonal distortion parameter α (see text). Symbols denote experimental data points—solid lines are theoretical curves using equations (2, 3, 4) and the quantum chemically computed g factors g || =2.31, g ⊥ =1.76 (see Table 1 ); dashed lines are calculated assuming isotropic g factors. Full size image where , and Γ zz couples the and components (along the c axis, perpendicular to the ab -plane IrO 2 layers [23] ) in the third term of equation (1) (see Methods for details). Experimental results are shown for v ||2 in Fig. 2a . The data comprise at T ≪ T N =240 K a group of overlapping resonances ( Fig. 2a , inset), possibly due to some distribution of internal fields in the sample. Though revealing some scatter, the AFR data follow approximately a parabolic dependence on h and, most importantly, they lie substantially above the curve corresponding to the free-electron Landé factor g e =2 (dashed line in Fig. 2a ). The experimental dependence can be reasonably well modelled with g || values of 2.3–2.45. The solid line in Fig. 2a is obtained by using g || =2.31, as derived from quantum chemistry calculations that will be discussed later on. Sizeable deviations to values >2 of g || is clear indication of the presence of low-symmetry, noncubic crystal fields. In the simplest approximation, that is, restricting ourselves to the Ir 4+ manifold, the anisotropic g factors in axial noncubic environment can be expressed up to the sign as [13] g || = g c =(2+2 k )cos 2 α −2sin 2 α and where k is a covalency reduction factor, α =(1/2) arctan parameterizes the deviation from octahedral symmetry, λ is the SOC constant and δ the Ir t 2g splitting. A plot for the dependence of the diagonal g factors on the distortion parameter α is shown in the inset to Fig. 2b . For simplicity, k =1 is for the moment assumed but smaller values of k do not bring qualitative changes. In cubic symmetry δ =0, α cub =35.26° and the g matrix is isotropic with . According to standard textbooks on ligand-field theory [24] , an elongation of the out-of-plane Ir-O bond induces a positive tetragonal splitting of the Ir t 2g levels, with δ >0 and α > α cub , whereas a bond compression yields δ <0 and α < α cub (see Fig. 1 ). As in Sr 2 IrO 4 the IrO 6 octahedra are substantially elongated in the z direction [23] , the g factors are expected to correspond to the case of positive splitting α > α cub , see the area to the right of the crossing point shown in the inset to Fig. 2b . It follows from the plot that g || <2, which obviously contradicts our AFR data for h || z [ Fig. 2a ]. The value g || =2.31 used to draw the curve connecting the open circles in Fig. 2a in fact corresponds to α =32.05°< α cub (see the inset in Fig. 2b ) and indicates that, despite the positive c -axis tetragonal distortion, a counterintuitive negative tetragonal splitting of the 5 d t 2g levels is present in Sr 2 IrO 4 . It should be noted that there is no Goldstone mode for finite in-plane magnetic fields. The canting angle depends in this case both on the strength of the DM interaction and the applied field. The two modes are and where and m is the in-plane ferromagnetic component of the effective moments. To first order in magnetic field, m can be expressed as which holds for weak fields where m remains small. The first term corresponds to the zero-field canting, arising from the DM interaction, while the second term shows how this canting evolves with increasing h ⊥ . Plots based on equations (3, 4) and the quantum chemically derived interaction parameters (see below) are displayed in Fig. 2b together with ESR data. Quantum chemistry calculations of g factors Results of ab initio quantum chemistry calculations for the g factors in Sr 2 IrO 4 and in the structurally related material Ba 2 IrO 4 are listed in Table 1 . Our computational scheme follows the prescription of Bolvin [27] and Vancoillie et al. [28] . It maps the matrix elements (MEs) of the ab initio Zeeman Hamiltonian onto the MEs of the effective pseudospin Hamiltonian , where μ , L and S are magnetic moment, angular-momentum and spin operators, respectively. The spin-orbit GS wave functions are computed either at the complete-active-space self-consistent-field (CASSCF) or multireference configuration-interaction (MRCI) level of theory [29] , as described in ref. 30 and using the MOLPRO quantum chemistry package [31] . All necessary angular-momentum MEs are calculated as well with MOLPRO (see Methods). In a first set of calculations, only the three t 2g orbitals at a given Ir site and five electrons were considered in the active space. The self-consistent-field optimization was carried out for the corresponding state. We use here the more convenient notations associated to O h symmetry, although the calculations were performed for the actual experimental geometry, with point-group symmetry lower than octahedral. Inclusion of SOC yields in this case a set of three Kramers doublets (KDs), see Table 1 . Table 1 g factors for Sr 2 IrO 4 and Ba 2 IrO 4 . Full size table Subsequently we performed calculations with larger active spaces, including also the Ir e g orbitals. One plus four ( 2 A 2g , 2 T 1g , 2 E g and 2 T 2g ) spin doublets, two spin quartets [ and ] and one spin sextet entered here the spin-orbit treatment. The orbitals were optimized for an average of all these terms. The effect of enlarging the active space to include terms in the reference wavefunction is in the range of 10%, in line with earlier semi-empirical estimates for 4 d 5 and 5 d 5 systems [15] , [16] , [17] , [18] . Most importantly, the calculations yield a negative tetragonal splitting of the Ir t 2g levels in Sr 2 IrO 4 , δ =−155 meV by MRCI, and positive t 2g splitting in Ba 2 IrO 4 (see Table 1 and Methods). Similar signs, negative in Sr 2 IrO 4 and positive in Ba 2 IrO 4 , but much larger magnitudes (≈0.7 eV) are found for the computed Ir e g splittings (not shown in Table 1 ). Taken together, the ESR and quantum chemistry results unequivocally point at an anomalous order of the split Ir 5 d levels in Sr 2 IrO 4 , related to the important role of the extended crystalline surroundings in generating low-symmetry fields that compete with ‘local’ distortions of the ligand cage. Similar effects were found by ab initio calculations on the 214 layered rhodate Sr 2 RhO 4 (ref. 32 ) and the 227 pyrochlore iridates [22] . In contrast, in Ba 2 IrO 4 , the stretch of the apical Ir-O bonds is strong enough [33] to overcome the longer-range electrostatics, turning the tetragonal t 2g positive again, as discussed in more detail in the following. Consequently, the structure of the tensor in Ba 2 IrO 4 is qualitatively different, with g ⊥ >2 and g || <2 (see Table 1 ), the ordering that one normally expects and encounters for elongated octahedra [13] . Exchange couplings from quantum chemistry To obtain ab initio quantum chemistry values for the inter-site effective magnetic couplings in Sr 2 IrO 4 (see equation (1)), we carried out additional calculations on larger clusters that incorporate two 5 d 5 sites. The two-octahedra cluster has C 2v symmetry (see Fig. 3 ), which implies a diagonal form for and in equation (1) (see Methods). 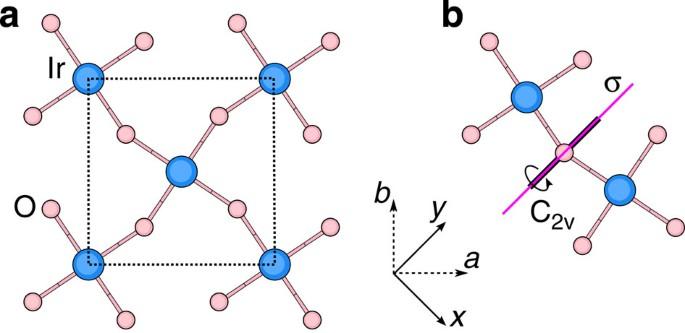Figure 3: Planar IrO2network in Sr2IrO4. (a) Coordination of the Ir site. Dashed lines show the boundaries of the crystallographic unit cell within a given IrO2layer. (b) The point-group symmetry of the [Ir2O11] block isC2v; associated symmetry elements are indicated in the figure. By one-to-one correspondence between the MEs of the ab initio Hamiltonian Figure 3: Planar IrO 2 network in Sr 2 IrO 4 . ( a ) Coordination of the Ir site. Dashed lines show the boundaries of the crystallographic unit cell within a given IrO 2 layer. ( b ) The point-group symmetry of the [Ir 2 O 11 ] block is C 2v ; associated symmetry elements are indicated in the figure. Full size image and the MEs of the effective spin Hamiltonian (1) in the basis of the lowest four spin-orbit states defining the magnetic spectrum of two NN octahedra, we can derive in addition to the g factors the strengths of the Heisenberg and anisotropic intersite couplings. In equation (6), is the scalar-relativistic Born-Oppenheimer Hamiltonian, describes spin-orbit interactions [30] and is the two-site Zeeman Hamiltonian. Diagonalization of the spin Hamiltonian (1) provides the expected singlet and three (split) triplet components | t x 〉, | t y 〉 and . Owing to the DM interaction, and are admixtures of ‘pure’ |0,0〉 and |1,0〉 spin functions. Our mapping procedure yields J ≈48 meV, somewhat lower than J values of 55–60 meV derived from experiment [9] , [34] , and a ratio between the DM and Heisenberg couplings D / J =0.25, in agreement with estimates based on effective superexchange models [12] , [35] , [36] and large enough to explain the nearly rigid rotation of magnetic moments that is observed when the IrO 6 octahedra revolve [37] , [38] . Ab initio results for the NN anisotropic couplings , also relevant for a detailed understanding of the magnetic properties of Sr 2 IrO 4 , are shown as well in Table 2 . In our convention the x axis is taken along the Ir-Ir link, that is, it coincides with the 〈110〉 crystallographic direction [23] , and z || c . We obtain Γ xx ≈Γ zz , which then allows to recast the Heisenberg and symmetric anisotropic terms in (1) as , with Γ xx =Γ zz =−Γ yy /2. Equally interesting, for no rotation of the IrO 6 octahedra and straight Ir-O-Ir bonds in Ba 2 IrO 4 , it is Γ yy and Γ zz which are approximately the same, providing a realization of the compass-Heisenberg model [36] , [39] since the DM coupling is by symmetry 0 in that case. Table 2 Nearest-neighbour magnetic couplings in Sr 2 IrO 4 . Full size table The two-site magnetic Hamiltonian (1) features in-plane symmetric-anisotropy couplings Γ xx and Γ yy , which were not considered in previous studies [12] , [26] . In the presence of two-sublattice order, terms containing these couplings cancel each other in the mean-field energy but they are in general relevant for pseudospin fluctuations and excitations. Using spin-wave theory and effective parameters derived from the quantum chemistry calculations, we nicely reproduce the correct GS and character of the modes, as shown in Fig. 2 . To reproduce the experimental zero-field gap, in particular, we used J , D and g -factor values as listed in Table 2 and a somewhat larger Γ zz parameter of 0.98 meV. To leading order, the dependence of and on h is linear, see equations (3, 4), and the slope is proportional to m . At low fields (≤1 T), m can be actually replaced with its field independent value [26] . Using the MRCI coupling constants, the first term in equation (5) then yields a moment m ≈0.12 μ B , in good agreement with the experiment [8] , [40] . The exact d -level order is of fundamental importance in TM oxides, dictating for instance the symmetry of the quasiparticle states in photoemission [10] , [32] , [41] and the nature of the magnetic ordering [42] , [43] . In 214 iridates specifically, it determines the various isotropic as well as anisotropic contributions to the magnetic exchange couplings [12] , [35] , [36] , [39] , the evolution of those magnetic interactions with strain [44] and/or pressure [19] and most likely the nature of the intriguing transition to a nonmagnetic phase in Sr 2 IrO 4 under high pressure [19] . Having established that in Sr 2 IrO 4 the d levels are inverted and that in the closely related Ba 2 IrO 4 they are not raises the question what actually drives the inversion. To address this, we performed an additional set of calculations, in which we change the charges around the reference IrO 6 octahedron. As a simple numerical experiment that preserves charge neutrality of the A 2 IrO 4 system, we assigned the 4 NN iridium sites (in-plane, see Fig. 4 ) the charge Q TM −2Δ q and the 8 closest A-site cations (out of plane) the valence Q A +Δ q . In a fully ionic picture, Q TM and Q A are 4+and 2+, respectively. However, since in our calculations the NN TM and A sites are not modelled as just formal point charges (see Methods), the actual valence states depart from their formal values, with larger ‘deviations’ for Q TM . The way we introduce Δ q in the computations is therefore by appropriately modifying the nuclear charge at the respective site. For variable Δ q , this interpolates linearly between nearby surroundings corresponding to 5 d 214 layered perovskites (with Δ q =0 and TM 4+ , A 2+ formal valence states) and their cuprate 214 equivalents (with Δ q =1, TM 2+ /A 3+ formal ionic charges and ‘normal’ order of the TM t 2g and e g levels [45] ). 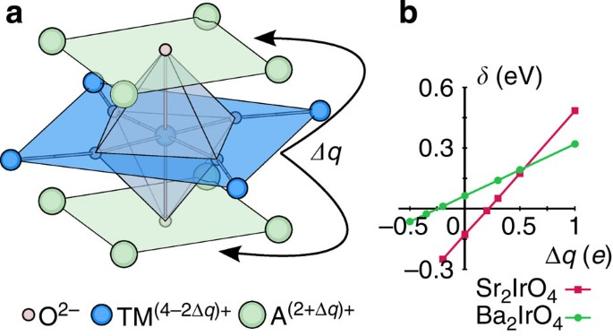Figure 4: Effect of interlayer charge imbalance in A2IrO4iridates. (a) The nearby surroundings of TM sites in A2TMO4-layered perovskites. In test calculations one can assign the adjacent (in-plane) TM ions the formal chargeQTM−2Δq, which is compensated by assigning the NN A sites the chargeQA+Δq. (b) Tetragonal crystal-field energy splitting betweent2gorbitals (δ) as a function of the charge redistribution Δqfor Sr2IrO4and Ba2IrO4. Figure 4: Effect of interlayer charge imbalance in A 2 IrO 4 iridates. ( a ) The nearby surroundings of TM sites in A 2 TMO 4 -layered perovskites. In test calculations one can assign the adjacent (in-plane) TM ions the formal charge Q TM −2Δ q , which is compensated by assigning the NN A sites the charge Q A +Δ q . ( b ) Tetragonal crystal-field energy splitting between t 2g orbitals ( δ ) as a function of the charge redistribution Δ q for Sr 2 IrO 4 and Ba 2 IrO 4 . Full size image As is illustrated in Fig. 4a , increasing Δ q amounts to moving positive charge from the IrO 2 plane to the adjacent A-O layers. The calculations show that upon moving charge in such a manner, the Ir t 2g splitting δ increases, see Fig. 4b . In other words, this redistribution of charge counteracts the level inversion in Sr 2 IrO 4 and further increases the already positive δ in Ba 2 IrO 4 . In Sr 2 IrO 4 the cubic-like j eff =1/2 limit occurs for Δ q =0.22. This effect can easily be understood: placing more positive charge out of the IrO 2 plane stabilizes the out-of-plane t 2g orbitals, corresponding to the ( yz , zx ) orbital doublet, and thus enhances δ . One can also do the opposite and drive Δ q negative. In this case more positive charge piles up in the IrO 2 plane, which one expects to lower the energy of the xy orbital singlet, thus enhancing the level inversion in Sr 2 IrO 4 . This is indeed what happens, see Fig. 4b . What is more, driving Δ q negative even causes a level inversion in Ba 2 IrO 4 , when Δ q −0.25. It is interesting to note that the slope of the δ versus Δ q lines in Sr 2 IrO 4 is much steeper than in Ba 2 IrO 4 , which is caused by the significantly smaller Ir–Ir distances in Sr 2 IrO 4 . From these test calculations it is clear that low-symmetry crystal fields associated to neighbours beyond the first ligand coordination shell, in particular, the highly charged Ir 4+ NNs, counteract the local tetragonal crystal field that is caused by the elongation of the IrO 6 octahedra in both Sr 2 IrO 4 and Ba 2 IrO 4 . In the case of Ba 2 IrO 4 the local distortion is still strong enough to overcome these longer-range effects but in Sr 2 IrO 4 , with a slightly smaller tetragonal distortion, the longer-range electrostatics wins, causing the observed level inversion. While the role of the high ionic charge of in-plane ions has been earlier invoked in the tetravalent Ru oxide compound Ca 2 RuO 4 (ref. 43 ) and in mixed-valence manganites [46] , we here explicitly prove it by combined ESR measurements and many-body ab initio calculations on structurally and chemically simpler systems in which additional complications arising from further distortions [43] , [47] or the presence of multiple TM valence states [46] are excluded. A reversed order of the Ir t 2g levels in Sr 2 IrO 4 has been also indirectly implied by fits of X-ray absorption [19] and X-ray magnetic scattering [37] , [48] spectra. As a more direct and more sensitive experimental technique to such details of the valence electronic structure and with back up from truly ab initio many-body calculations, ESR now provides irrefutable evidence for such physics. The numerical ‘experiment’ outlined in Fig. 4 further shows that at the heart of this effect is not the intersite exchange, as assumed in ref. 19 , and not the t 2g - e g orbital hybridization invoked in ref. 48 , but basic interlayer electrostatics. We have, in sum, provided an integrated picture on the d -level structure and magnetic anisotropies in Sr 2 IrO 4 , a prototype spin-orbit driven magnetic insulator. Both the single-site tensor and intersite effective exchange interactions are analysed in detail. To access the latter, we build on an earlier computational scheme for deriving intersite matrix elements in mixed-valence spin-orbit coupled systems [49] . While the ratio D / J of the antisymmetric Dzyaloshinskii-Moriya and isotropic Heisenberg couplings is remarkably large in Sr 2 IrO 4 and concurs with an in-plane rotation pattern of the Ir magnetic moments that follows nearly rigidly the staggered rotation of the IrO 6 octahedra [37] , [38] , the most prominent symmetric anisotropic terms are according to the quantum chemistry data in-plane, perpendicular to the Ir-Ir links. The structure of the tensor, as measured by ESR and computed with first-principles electronic-structure methods, is such that and distinctly indicates a negative tetragonal-like splitting of the Ir t 2g levels, in spite of sizable positive tetragonal distortions in Sr 2 IrO 4 . We further observe that a much stronger tetragonal distortion in Ba 2 IrO 4 renders the tetragonal d -level splitting positive and g || < g ⊥ . The interesting situation arises that nevertheless the magnitude of the Ir t 2g splitting is largest in Sr 2 IrO 4 . The d -level inversion in Sr 2 IrO 4 and the surprisingly small splitting in Ba 2 IrO 4 have to do with the way the positive ionic charge is distributed between adjacent Ir 4+ O 2 and A 2+ O layers, having in contrast to the 214 cuprate superconductors, for example, more positive charge in the TM-O planes. This almost compensates the ‘local’ tetragonal field arising from the z axis elongation of the IrO 6 octahedra in Ba 2 IrO 4 and overcompensates it in Sr 2 IrO 4 . The subtle interplay between local distortions of the O ligand cage and additional uniaxial fields associated with the anisotropic extended surroundings opens new perspectives on strain [44] and pressure [19] experiments in square-lattice iridates, for example, in connection to the spin-flop transition earlier predicted in Sr 2 IrO 4 (refs 12 , 36 ). It also opens up the perspective of manipulating this way the d -level ordering in oxide heterostructures with highly charged, trivalent and tetravalent species. Compounds with tetravalent species within the TM-O 2 layers, in particular, given the nonpolar character of the quasi 2D sheets, provide ideal playgrounds to explore the mechanism of d -level ordering pointed out here since that will not be hindered by ‘interface’ charge redistribution and structural reconstruction occuring in polar heterostructures from polar discontinuities [50] , [51] . A recent experimental realization of such mixed, tetravalent/divalent TM-oxide interfaces is for example the SrRuO 3 /NiO interface [52] , one system that requires in this respect closer theoretical examination. Single-site magnetic properties The g factors were obtained by computations on clusters which contain one central IrO 6 octahedron, the four NN IrO 6 octahedra and the nearby ten Sr/Ba ions. The solid-state surroundings were modelled as a large array of point charges fitted to reproduce the crystal Madelung field in the cluster region. To obtain a clear picture on crystal-field effects and spin-orbit interactions at the central Ir site, we cutoff the magnetic couplings with the adjacent Ir ions by replacing the tetravalent open-shell d 5 NNs with tetravalent closed-shell Pt 4+ species. This is a usual procedure in quantum chemistry studies on TM systems, see for example, refs 42 , 45 , 53 , 54 , 55 , 56 . We used energy-consistent relativistic pseudopotentials and valence basis sets of quadruple-zeta quality supplemented with f polarization functions for the central Ir ion [57] and all-electron triple-zeta basis sets for the six adjacent ligands [58] . For the TM NNs, we applied energy-consistent relativistic pseudopotentials and triple-zeta basis functions [57] along with minimal atomic-natural-orbital basis sets [59] for the Os coordinating those TM sites but not shared with the central octahedron. The Sr and Ba species were modelled by divalent total-ion effective potentials supplemented with a single s function [60] . All O 2 p and metal t 2g electrons at the central octahedron were correlated in the MRCI calculations. The latter are performed with single and double substitutions with respect to the CASSCF reference (for technicalities, see refs 61 , 62 ), which is referred to as MRCISD. To separate the metal 5 d and O 2 p valence orbitals into different groups, that is, central-octahedron and adjacent-octahedra orbitals, we used the Pipek-Mezey localization module [63] available in MOLPRO. The computations with hypothetical ( Q TM −2Δ q ) and ( Q A +Δ q ) ionic charges at the TM and Sr/Ba sites next to the reference Ir ion were carried out as frozen-orbital multideterminant calculations (also referred to as CASCI) with three Ir t 2g and five electrons in the active space and orbitals optimized for Δ q =0. The spin-orbit treatment was performed according to the procedure described in ref. 30 . In a first step, the scalar relativistic Hamiltonian is used to calculate correlated wavefunctions for a finite number of low-lying states, either at the CASSCF level or at the MRCI level. In a second step, the spin-orbit part is added to the initial scalar relativistic Hamiltonian, matrix elements of the aforementioned states are evaluated for this extended Hamiltonian and the resulting matrix is finally diagonalized to yield SO wavefunctions. The g factors were computed following the scheme proposed by Bolvin [27] and Vancoillie et al. [28] (for alternative formulations, see, for example, ref. 64 ). For the KD GS , the Abragam-Bleaney tensor [13] , [65] , G = gg T can be written in matrix form as where The MEs of are here provided by MOLPRO while those of are derived using the conventional expressions for the generalized Pauli matrices : G is next diagonalized and the g factors are obtained as the possitive square roots of the three eigenvalues. The corresponding eigenvectors specify the rotation matrix to the main magnetic axes. In our case, the magnetic z axis is along the crystallographic c coordinate, while x and y are ‘degenerate’ and can be any two perpendicular directions in the ab plane. To cross-check the g -factor values computed with our subroutine, we further performed g -factor calculations using the module available within the ORCA quantum chemistry package [66] . We applied all-electron DKH (Douglas-Kroll-Hess) basis sets of triple-zeta quality for the TM ions [67] , triple-zeta basis functions for the ligands of the central octahedron [58] and double-zeta basis functions for additional Os at the NN octahedra [58] . Dynamical correlation effects were accounted for by N -electron valence-state second-order perturbation theory (NEVPT2) [68] , [69] . CASSCF and NEVPT2 results are listed in Table 3 , for both Sr 2 IrO 4 and Ba 2 IrO 4 . It is seen that the data in Tables 1 and 3 compare very well and indicate the same overall trends. Table 3 Ir t 2g splittings and g factors for Sr 2 IrO 4 and Ba 2 IrO 4 . Full size table Superexchange interactions in Sr 2 IrO 4 NN magnetic coupling constants were obtained for Sr 2 IrO 4 by calculations on an embedded cluster that includes two IrO 6 octahedra as magnetically active units. As for the calculation of single-site magnetic properties, to accurately describe the charge distribution in the immediate neighbourhood, the adjacent IrO 6 octahedra (six) and the closest Sr 2+ ions (16) were also incorporated in the actual cluster. We used energy-consistent relativistic pseudopotentials along with quadruple-zeta basis sets for the valence shells of the two magnetically active Ir ions [57] , all-electron quintuple-zeta basis sets for the bridging ligand [58] and triple-zeta basis functions for the other Os associated with the two reference octahedra [58] . We further employed polarization functions at the two central Ir sites and for the bridging anion, namely 2 Ir f and 4 O d functions [57] , [58] . Additional ions defining the NN octahedra, the nearby Sr 2+ species and the farther crystalline surroundings were modelled as in the single-site study, see above. For two adjacent magnetic sites, the manifold entails nine singlet and nine triplet states. The CASSCF optimization was carried out for an average of these nine singlet and nine triplet eigenfunctions of the scalar relativistic Hamiltonian . In the subsequent MRCI treatment, only the Ir t 2g and the O 2 p electrons at the bridging ligand site were correlated. Results in good agreement with the experimental data were recently obtained with this computational approach for related 5 d 5 iridates [21] , [70] . Diagonalization of the Hamiltonian in the basis of the lowest nine singlet and nine triplet states provides a total of 36 spin-orbit-coupled eigenfunctions, namely, four , eight , eight and sixteen states. In the simplest picture, the lowest four roots imply either singlet or triplet coupling of the spin-orbit j eff =1/2 (or, more generally, pseudospin =1/2) on-site objects and are separated from higher-lying states by a gap of 0.5 eV, much larger than the strength of the intersite exchange. It is this set of lowest four spin-orbit MRCI roots that we map onto the eigenstates of the effective two-site (pseudo)spin Hamiltonian (1). The Zeeman interaction shows up on the quantum chemistry side as , where and are transformed to the spin-orbit-coupled basis using the spin-orbit wavefunctions as unitary transformation matrix. MEs of the ab initio model Hamiltonian are shown in Table 4 . Diagonal components show the energies of the zero-field states, while the off-diagonal MEs describe the coupling to magnetic field. Table 4 Matrix elements of the ab initio spin-orbit Hamiltonian. Full size table For the experimentally determined crystal structure of Sr 2 IrO 4 (ref. 23 ), the two-octahedra [Ir 2 O 11 ] cluster displays C 2 v symmetry. Having the x axis along the 〈110〉 crystallographic direction [23] and z || c , the effective anisotropic couplings read D =(0,0, D ), for Ir-Ir links along x and for Ir-Ir links along y , with Γ xx +Γ yy +Γ zz =0. The uniform and staggered components of the tensor take for individual Ir sites the following form : g zz = g || while g xx and g yy are directly related to g ⊥ but not restricted to be equal due to the lower symmetry of the two-octahedra cluster as compared with the IrO 6 unit. To solve now the actual problem, we need to transform the effective spin Hamiltonian (1) to the same form as the ab initio Hamiltonian shown in Table 4 , that is, diagonal in zero magnetic field. The result of such a transformation is shown in Table 5 . Direct correspondence between homologous MEs in the two arrays yields a set of eight independent equations that finally allow to derive hard values for all effective coupling constants that enter expression (1). While the results for the intersite exchange interactions in (1) and (10,11) are shown in Table 2 , the -tensor data obtained from the two-octahedra calculations are g xx =1.64, g yy =1.70, g zz =2.31 and g xy =0.02. The way the additional parameters introduced in Table 5 are defined is explained in Table 6 . The intermediate steps followed to arrive to the matrix form provided in Table 5 are outlined in Supplementary Tables I–III and the Supplementary Methods . Table 5 Matrix elements of the effective spin Hamiltonian. Full size table Table 6 Notations used for anisotropic exchange coupling parameters in Sr 2 IrO 4 . Full size table Spin-wave calculations For understanding all details of the ESR spectrum, we carried out a spin-wave analysis using the Hamiltonian (1) and a site-factorized variational GS wave function where for each sublattice index L ∈ { A , B }, For the 2D unit cell displayed in Fig. 3a , D 2 d symmetry is considered. The spin components of the GS configuration depend on the α L and variational parameters as For magnetic fields parallel to the c axis, the GS energy only depends on the parameters α A = α B = α and . is the angle between neighbouring in-plane spins and α describes how much the spins are tilted away from the c axis. For α = π /2 the spins are lying within the ab plane, while α =0 corresponds to the fully polarized high-magnetic-field case. The GS energy is minimized when For zero field we find that α =0, the spins are confined to the ab plane (that is, to the IrO 2 layer) and the angle is controlled by the strength of D . is not affected by fields along the c axis while α changes smoothly from π /2 to 0 with increasing the field strength. The two magnons characteristic for spin-1/2 antiferromagnets are related to states orthogonal to and . The 4 × 4 Hamiltonian defining these magnons can be derived by using the well-known Holstein-Primakoff approach and diagonalized through a Bogoliubov transformation. For h || c , the two spin-wave modes are the gapless v ||1 =0 Goldstone mode, corresponding to U(1) symmetry breaking, and the gapped mode given by (2). When the magnetic field lies in the ab plane, the z component of Ir spins remains zero (with α = π /2) and the GS energy only depends on the angle : For simplicity, we select x for the direction of the magnetic field. The result is, however, independent of how this choice is made as there is no anisotropy within the ab plane. An infinitesimally small in-plane field fixes the direction of uniform magnetization as . At finite field both modes thus become gapped. To determine the uniform magnetization m one needs to minimize equation (21), which to leading order in magnetic field leads to equation (5). The first term of equation (5) corresponds to the zero-field moment, which arises due to the canting induced by the DM interaction. This ferromagnetic order-parameter is further enhanced in finite h ⊥ field. As long as h ⊥ is small equation (5) remains valid. As discussed in the main text, in low fields, m can be approximated by its field independent value [26] . Using the quantum chemically derived interaction parameters (see Table 2 ), we then find m ≈0.12 μ B , in good agreement with recent experiments [8] , [40] . Yet the zero-field gap comes out too large as compared to experiment. A good fit can nevertheless be reached with J , D and g values as obtained in the MRCI treatment and by increasing Γ zz from 0.42 to 0.98 meV. How to cite this article: Bogdanov, N. A. et al. Orbital reconstruction in nonpolar tetravalent transition-metal oxide layers. Nat. Commun. 6:7306 doi: 10.1038/ncomms8306 (2015).